Nlrc3 signaling is indispensable for hematopoietic stem cell emergence via Notch signaling in vertebrates Hematopoietic stem and progenitor cells generate all the lineages of blood cells throughout the lifespan of vertebrates. The emergence of hematopoietic stem and progenitor cells is finely tuned by a variety of signaling pathways. Previous studies have revealed the roles of pattern-recognition receptors such as Toll-like receptors and RIG-I-like receptors in hematopoiesis. In this study, we find that Nlrc3 , a nucleotide-binding domain leucine-rich repeat containing family gene, is highly expressed in hematopoietic differentiation stages in vivo and vitro and is required in hematopoiesis in zebrafish. Mechanistically, nlrc3 activates the Notch pathway and the downstream gene of Notch hey1 . Furthermore, NF-kB signaling acts upstream of nlrc3 to enhance its transcriptional activity. Finally, we find that Nlrc3 signaling is conserved in the regulation of murine embryonic hematopoiesis. Taken together, our findings uncover an indispensable role of Nlrc3 signaling in hematopoietic stem and progenitor cell emergence and provide insights into inflammation-related hematopoietic ontogeny and the in vitro expansion of hematopoietic stem and progenitor cells. Hematopoietic stem and progenitor cells (HSPCs) have the extraordinary ability to both self-renew and generate all the known blood cell lineages. In all vertebrate embryos, HSPCs arise from the hemogenic endothelium (HE) of the dorsal aorta (DA) during a transitory developmental process as the hemogenic endothelial to hematopoietic transition (EHT). Previous studies have provided a more comprehensive understanding of the signaling pathways that orchestrate HSPCs emergence. Pattern-recognition receptors (PRRs), including Toll-like receptor 4 ( TLR4 ) and RIG-I-like receptors (RLR) [1] , [2] , play essential roles in embryonic HSPC production. However, it remains largely unknown what the roles and mechanisms of the nucleotide-binding oligomerization domain (NOD)-like receptors (NLRs) are in this process. It is known, however, that NLRs function as sensors of the innate immune system and regulators of cytokine secretion, which are important for vertebrate hematopoiesis. Nlrc3 , an intracellular member of the NLR family, has been reported to be highly expressed in various immune cells [3] , [4] . In mammals, Nlrc3 has been shown to be a negative regulator of numerous cellular populations, such as macrophages, dendritic cells (DCs), and T lymphocytes, and has also been shown to be involved in the host innate immune response to intracellular DNA and DNA viruses through NF-kB signaling [5] , [6] , [7] , [8] , [9] . Furthermore, Nlrc3 deficiency has been shown to increase the expression of proinflammatory cytokines, including interleukin-1β ( il1b ), il6 , il12 and tumor-necrosis factor a ( TNF-α ) in lipopolysaccharide-induced macrophages [7] . In teleost, emerging evidence has suggested the regulatory roles of piscine NLRC3 -like genes in pathogen infections and the production of proinflammatory cytokines [10] , [11] . Among these diverse biological functions that may affect homeostasis or disease pathogenesis, the explicit role of Nlrc3 in HSPCs, particularly in embryonic stages, remains poorly understood. Canonical Notch signaling is essential in the regulation of definitive HSPCs [12] . The emergence of the hemogenic endothelium (HE), from which definitive HSPCs are derived, is concomitant with arterial differentiation. Notch has been shown to be responsible for the loss of arterial identity [13] , [14] . In particular, proinflammatory factors such as tnfa [15] , interferon-gamma ( IFN-γ ) [16] , and il6 [17] have been reported to be associated with Notch in regulating HSPCs. However, the regulatory relationship between Nlrc3 , one of the PRRs involved in regulating these factors, and Notch remains undocumented. Moreover, among the ligands and receptors of Notch signaling, the Hey genes, which are helix-loop-helix transcription factors, such as Hey2 , act synergistically during all stages of arterial establishment [18] . Although it has been reported that Hey1 is involved in vascular development, little is known about its role in HSPC emergence [19] , [20] . The transcription factors of the nuclear factor k-light-chain enhancer of the activated B core (NF-kB) family serve as the master controllers of the inflammatory response, and the conserved NF-kB–Notch pathway is essential in HSPC emergence [1] , [21] . NLR proteins such as NOD1 , NOD2 , and NLRP3 can positively alter the activation of NF-kB in response to peptidoglycan stimulation [22] , [23] , [24] , [25] , but Nlrc3 has been reported to be an inhibitor of NF-kB through modulation of the ubiquitination of TRAF6 [7] , which has been shown to suppress the expansion of HSPCs in the fetal liver [26] . These results prompted us to hypothesize that Nlrc3 might play critical roles in vertebrate embryonic hematopoiesis through interacting with NF-kB. In this study, we delineated the functional roles of Nlrc3 signaling in the HSPC emergence in various systems, including published data of single-cell RNA-seq (scRNA-seq) and the embryonic stem cell (ESC) differentiation system in vitro [27] , [28] , [29] , [30] , as well as in zebrafish and mouse models in vivo. Mechanistically, we found that during the embryonic stage, NF-kB regulates Nlrc3 through transcriptional activity, and Nlrc3 acts upstream of Notch and Hey1 , these factors forming an essential axis of NF-kB- Nlrc3 -Notch- Hey1 is indispensable for HSPCs emergence. Overall, our study revealed an undiscovered role of Nlrc3 signaling in the generation of embryonic HSPCs under nonpathogenic conditions and emphasizes the vital role of pattern recognition receptor signals in the formation of HSPCs during development. NLRC3 is highly expressed during vertebrate HSPC development in vivo and in vitro Previous studies in vertebrate embryos uncovered the role of inflammatory signaling in HSPC emergence. To explore the potential pathways involved in hematopoietic ontogeny and differentiation in this stage, we screened the dynamic expression of NLR family genes and other genes related to inflammation in the published scRNA-seq data in vertebrates’ embryos during HSPC development. In a data profiling caudal hematopoietic tissue (CHT) of zebrafish at 3.5 and 4.5 days postfertilization (dpf) [27] , Compared to many other NLR family paralogs, including nlrp1 , nlrp3 , nlrc3l , nlrc5 , nlrc6 , nlrx1 and nlrp16 , the expression of nlrc3 is relatively higher in the ECs and HSPCs subpopulations (Fig. 1a ). To further investigate the expression of nlrc3 in mammalian models, we analyzed published single-cell transcriptomic data profiling mouse embryo from 9.5 days post coitus (dpc) to 11.5 dpc [28] . Comparison of Aorta Gonad Mesonephros (AGM)–derived HSPCs and fetal liver (FL)-derived HSPCs with venous endothelial cells (VECs), arterial endothelial cells (AECs), pre-hemogenic endothelial cells (pre-HECs) and hemogenic endothelial cells (HECs), the expression of Nlrc3 increases with hematopoietic maturation, especially when comparing HECs with HSPCs, which is the stage that hemogenic endothelial to hematopoietic transition (EHT) occurs (Fig. 1b ). And the expression of Nlrc3 is not only highly expressed among the NLR family genes but also like that of Tlr4 , which has been reported to be involved in the regulation of HSPC development [1] . Furthermore, in the latest single-cell transcriptome map of human hematopoietic tissues from the first trimester [29] , the expression trend of NLRC3 was also validated to be enriched in venous endothelium (VE), arterial endothelium (AE), hemogenic endothelium (HE), HSCs and HPCs which are defined as Non-HSCs (Fig. 1c ), especially the differentiation stage from HE to HSCs. Fig. 1: NLRC3 is highly expressed during vertebrates HSPC development. a Schematic paradigm of zebrafish caudal hematopoietic tissue (CHT) tissue for single-cell RNA-seq (scRNA-seq) profiling. Bubble plot of scRNA-Seq data demonstrating the expression of nucleotide-binding domain leucine-rich repeat (NLR) family members, including Nlrc3 and related inflammatory genes in the clusters of endothelial cells (ECs) and Hematopoietic stem and progenitor cells (HSPCs). b Schematic paradigm of mouse embryonic Aorta Gonad Mesonephros (AGM) for scRNA-seq profiling. Bubble plot of scRNA-Seq data demonstrating the expression of NLR family members, including Nlrc3 and related inflammatory genes in the clusters of venous endothelial cells (VECs), arterial endothelial cells (AECs), pre-hemogenic endothelial cells (pre-HECs), hemogenic endothelial cells (HECs), HSPCs, fetal liver (FL)-derived HSPCs. c Schematic paradigm of human embryonic AGM for scRNA-seq profiling. Bubble plot of scRNA-Seq data demonstrating the expression of NLR family members, including NLRC3 and inflammatory genes in the clusters of venous endothelium (VE), arterial endothelium (AE), hemogenic endothelium (HE), HSPCs and Non-HSCs. Illustrations created with BioRender.com. Source data are provided as a Source Data file. Full size image Although rather in the primitive stage, the hematopoietic differentiation system using embryonic stem cells (ESCs) is a convenient research model that simulates and observes the in vivo embryonic hematopoiesis, in which cells gradually differentiate into the mesoderm, HE, and HSPCs stages, and are accompanied by specific different molecular markers at different stages [31] , [32] . To further verify the expression of Nlrc3 in vitro, we compared FL- and bone marrow (BM)-derived HSPCs with HSC-like cells derived from mouse ESCs (Supplementary Fig. 1a ) [30] . Differential gene expression analysis using RNA-seq revealed that among the NLR family genes, Nlrc3 expression was highly enriched with the expression of genes that have been reported to regulate the emergence of HSCs, including Tlr4 [1] and IFN-γ [16] (Supplementary Fig. 1b ). We further validated our results by employing the in vitro HSC-like cell differentiation system using human embryonic stem cells (hESCs) (Supplementary Fig. 1c ). We examined the dynamic change of NLRC3 during the 12-day hematopoietic differentiation process by qPCR and found that compared with day 0, the expression of NLRC3 gradually increased along with the hematopoietic differentiation from hESCs (Supplementary Fig. 1d ). Moreover, we isolated cells from different stages (hESCs at Day 0, CD309 + mesoderm cells at Day 3, CD31 + CD34 + HE cells at Day 6, CD43 + HSPCs cells at Day 9, and CD45 + HSPCs at Day 12). Our qPCR results showed that, compared with undifferentiated hESCs, the expression of NLRC3 in HE was significantly increased by approximately 300-fold and was even higher in CD43 + and CD45 + HSPCs (Supplementary Fig. 1e ). TLR4 and NLPR3 , which have been reported to be regulators of HSPCs emergence and differentiation, showed a similar trend to NLRC3 (Supplementary Fig. 1f, g ). Overall, these results suggest that NLRC3 was highly expressed during embryonic HSPC development in vivo and vitro and might play an important role in HSPC emergence in vertebrates. Nlrc3 signaling is indispensable for HSPC production in zebrafish To investigate whether nlrc3 signaling is required for in vivo HSPC emergence, we synthesized probes from the full-length mRNA of nlrc3 and utilized them to observe the in-situ expression of nlrc3 in zebrafish at different developmental stages. The WISH experiment demonstrated that nlrc3 was expressed from the 1-cell stage and, importantly, showed specific expression in the AGM region of zebrafish at 24–28hpf, which coincides with the onset of HSPC generation. There was also a high expression of nlrc3 at 72hpf in the CHT region, which follows a similar spatiotemporal expression pattern as HSPC generation, indicating that nlrc3 may be involved in the development of HSPCs (Supplementary Fig. 2a ). By co-staining with arterial endothelial-specific markers dlc and efnb2 (Supplementary Fig. 2b, c ), hematopoietic stem/progenitor cell-specific markers runx1 and cmyb (Supplementary Fig. 2d, e ), we found that co-staining nlrc3 with these probes can effectively enhance the expression of HE and HSPCs. These results suggest that nlrc3 may be involved in the regulation of this process in zebrafish. In order to validate this hypothesis, loss-of-function experiments were performed using zebrafish with a targeted Morpholino (MO) (Supplementary Fig. 3a ). We observed the floor of the DA region in Tg ( runx1 :EGFP/ kdrl :mCherry) double-transgenic embryos at 28 hpf by confocal microscopy, runx1 is a conserved HSPC marker and kdrl is a vascular endothelial-specific marker, the runx1 + kdrl + cells signifies HSPCs occurs through the hemogenic endothelial (HE) to hematopoietic transition (EHT) process is this time point, and the number of runx1 + kdrl + HSPCs of morphants was significantly lower than that in control embryos (Fig. 2a, b ). By using the Tg( cmyb :EGFP/ kdrl :mCherry) double-transgenic line at 48 hpf, cmyb is another conserved HSPC marker, we found that the number of cmyb + kdrl + HSPCs of morphants within the ventral wall of the dorsal aorta (VDA) markedly decreased in nlrc3 morphants (Fig. 2c, d ). Tg ( CD41 : GFP), which is a well-established transgenic line with HSPC expansion in the CHT, also had reduced expression in morphants at 72 hpf (Fig. 2e, f ). Furthermore, we performed whole-mount in situ hybridization (WISH) to measure the expression of runx1 and cmyb , which are nascent HSPC markers at early developmental stages, and found that the expression of runx1 and cmyb was significantly reduced at 28 hpf and at 36 hpf, respectively, in the aortic floor of nlrc3 morphants compared with their wild-type siblings (Fig. 2g, j ). To further demonstrate the role of nlrc3 in HSPC emergence, we generated nlrc3 mutant by the CRISPR/Cas9, 29 bp base is knocked out in homozygotes (Supplementary Fig. 2b, c ). The expression of nlrc3 was abrogated in mutants at the site of HSPC occurrence at 24–36 hpf (Supplementary Fig. 3d, e ). Consistent with previous results, the expression of runx1 and cmyb was decreased in mutants by WISH at 28 hpf and 36 hpf, respectively (Fig. 2g–j ). With this mutant, we also validated the downregulation of hematopoietic markers and nlrc3 at 28 hpf by qPCR (Fig. 2k ). The similar phenotype between morphants and mutants allows for the experimental design to be tailored based on specific needs. To obtain more comprehensive evidence, we examined gata2b , a critical early hematopoietic marker [12] . Through qPCR, we found a downregulation of gata2b in the mutant at 28 hpf. Therefore, we synthesized the full-length mRNA of gata2b and overexpressed it. The reduction in runx1 at 28hpf and cmyb at 36 hpf due to nlrc3 deficiency was partially restored by the rescue of gata2b (Supplementary Fig. 3f, g ). This result was also confirmed by qPCR analysis (Supplementary Fig. 3h ). These results indicated that nlrc3 was required for HSPC emergence and expansion. Fig. 2: Nlrc3 signaling is indispensable for HSPC production in zebrafish. a , b Confocal imaging showing the number of hemogenic endothelium and emerging HSPCs in runx1 + kdrl + cells from Tg ( runx1 :EGFP/ kdrl :mCherry) embryos at 28 hpf in the AGM (white arrowheads) in control embryos and nlrc3 morphants with quantification ( b ). **** P < 0.0001, n = 11, 10 embryos. c , d Confocal imaging showing the number of cmyb + kdrl + cells in Tg ( cmyb :EGFP/ kdrl :mCherry) embryos at 48 hpf in the AGM (white arrowheads) in control embryos and nlrc3 morphants with quantification ( d ). **** P < 0.0001, n = 10, 9 embryos. e , f Confocal imaging showing the number of HSPCs in Tg ( CD41 :GFP) embryos at 72 hpf in the CHT (white arrowheads) in control embryos and nlrc3 morphants with quantification ( f ). **** P < 0.0001, n = 9, 13 embryos. g , h Expression of the HSPC marker runx1 in nlrc3 morphants and mutants in the AGM region at 28 hpf by whole mount in situ hybridization (WISH) (black arrowheads) with quantification ( h ) **** P < 0.0001, n = 18, 32, 21 embryos. i , j Expression of the HSPC marker cmyb in nlrc3 morphants and mutants in the region of AGM and CHT at 36 hpf by WISH (black arrowheads) with quantification ( j ) **** P < 0.0001, n = 25, 37, 18 embryos. k Expression of nlrc3 and the HSPC genes runx1 , cmyb in control embryos and nlrc3 morphants at 28 hpf by qPCR. * P = 0.0462, *** P = 0.0006, 0.0010, n = 3 biological replicates. Error bars, mean ± s.d., **** P < 0.0001, by using two-tailed, unpaired Student’s t -test in ( b , d , f , k ), one-way ANOVA – Sidak test in ( h , j ). For the box plots in ( b , d , f , h , j ), box limits extend from the 25th to 75th percentile, while the middle line represents the median. Whiskers extend to the largest value no further than 1.5 times the inter-quartile range (IQR) from each box hinge. Scale bars, 100 μm in ( a , c , e , g , i ). Illustrations created with BioRender.com. Source data are provided as a Source Data file. Full size image To further evaluate the effect of nlrc3 on hematopoietic differentiation, we examined the expression of rag1 , which specifically indicates the differentiation capability of HSPCs for T cell lineages. WISH results showed that rag1 expression was markedly reduced in both morphants and mutants (Fig. 3a ). A similar phenotype was observed in Tg ( lck :EGFP) transgenic morphants at 120 hpf (Fig. 3b ), while lymphoid genes, including ikaros , rag1 , lck , and il7r , were downregulated in mutants, as assessed by qPCR (Fig. 3c ). However, the expression of the thymic epithelial cell marker foxn1 was normal (Fig. 3a ), suggesting that T-cell defects in these deficient embryos resulted from early HSPC defects. The expression of gata1a , an erythrocyte-specific marker, was decreased in the posterior blood island (PBI) and trunk regions of morphants at 36 hpf and 96 hpf, respectively (Supplementary Fig. 4a , Fig. 3d ), which was further verified by qPCR analysis in mutants (Fig. 3e ). We also examined the phenotypes of Tg ( lcr :EGFP) and Tg ( gata1a :DsRed) transgenic morphants at 60 hpf (Supplementary Fig. 4b, c ). These two transgenic lines are capable of tracking erythrocytes in blood vessels, and the results strongly suggest that nlrc3 signaling is essential for definitive erythropoiesis. Myeloid lineage differentiation was also impaired in mutants, as assayed by mpx at 96 hpf and l-plastin at 120 hpf by WISH (Fig. 3f , Supplementary Fig. 4f ). Similar phenotypes were assessed in Tg ( mpx :EGFP) and Tg ( lyz :DsRed) transgenic morphants as the neutrophil marker at 60 hpf and 72 hpf, respectively, in the CHT region (Supplementary Fig. 4d, e ), and the expression of myeloid-lineage genes in mutants at 96 hpf was found to be decreased by qPCR (Fig. 3g ). These results indicated that HSPC differentiation was impaired when nlrc3 signaling was disturbed. Fig. 3: Nlrc3 signaling is imperative for HSPC differentiation in zebrafish. a Expression of the lymphoid marker rag1 in nlrc3 morphants and mutants and the thymic epithelial cell marker foxn1 in the thymus of control embryos, nlrc3 morphants, and mutants at 96 hpf (black arrowheads). b Snapshot of lck + cells in Tg ( lck :EGFP) embryos in the thymus of control embryos and nlrc3 morphants at 5 dpf (white arrowheads). c Expression of nlrc3 and the lymphoid genes ikaros , rag1 , lck , and il7r in control embryos and nlrc3 morphants at 96 hpf by qPCR. * P = 0.0229, 0.0197, *** P = 0.0009. d Expression of the erythroid marker gata1a in control embryos and nlrc3 morphants by WISH at 96 hpf (black arrowheads). e Expression of nlrc3 and the erythroid gene gata1a in control embryos and nlrc3 morphants at 96 hpf by qPCR. ** P = 0.0011. f Expression of the myeloid marker mpx in control and nlrc3 morphants by WISH at 120 hpf (black arrowheads). g Expression of nlrc3 and the myeloid gene ikaros, l-plastin, pu.1, lyz , and csf1a in control embryos and nlrc3 mutants at 96 hpf by qPCR. * P = 0.0178, 0.0197, ** P = 0.0049, 0.0011, *** P = 0.0007, 0.0003. h Expression of nlrc3 and the HSPC genes runx1 and cmyb in control, nlrc3 morphants, and nlrc3 morphants with overexpression of nlrc3 mRNA at 30 hpf by qPCR. * P = 0.0286, 0.0272, 0.0158, ** P = 0.0040, 0.0047, 0.0068. i Expression of the HSPC marker runx1 in control embryos, nlrc3 morphants, and nlrc3 morphants with overexpression of nlrc3 mRNA at 48 hpf by WISH (black arrowheads). j Expression of the lymphoid marker rag1 in control embryos, nlrc3 morphants, and nlrc3 morphants with overexpression of nlrc3 mRNA at 96 hpf by WISH (black arrowheads). Error bars, mean ± s.d., * P < 0.05, ** P < 0.01, *** P < 0.001, **** P < 0.0001, the exact p -values mentioned above are listed from left to right, by using two-tailed, unpaired Student’s t -test in ( c , e , g ). Two-way ANOVA with Tukey’s post hoc test in ( h ). n = 3 biological replicates. Scale bars, 100 μm in ( a , b , d , f , i , j ). Illustrations created with BioRender.com. Source data are provided as a Source Data file. Full size image To determine if nlrc3 was sufficient for embryonic hematopoiesis, we synthesized nlrc3 mRNA for rescue experiments. The decreased expression of runx1 at 48 hpf and rag1 at 96 hpf could be rescued by overexpression of nlrc3 mRNA, as assessed by WISH, and qPCR also validated this trend at 30 hpf (Fig. 3h–j ). These results demonstrated that HSPC defects in nlrc3 -deficient embryos were specific. To further examine the role of nlrc3 in the first wave of hematopoiesis, which is generally called the “primitive” wave, we performed WISH to measure the expression of gata1a at 26 hpf (Supplementary Fig. 5a ). qPCR of gata1a at 30 hpf verified this phenotype, confirming that nlrc3 signaling may not impact primitive erythropoiesis (Supplementary Fig. 5b ). However, the expression of mpx was decreased at 24 hpf, as measured using WISH (Supplementary Fig. 5c ), indicating that the development of primitive neutrophils depended on nlrc3 signaling. Additionally, the expression of mfap4 , a specific marker of macrophages, was reduced in nlrc3 -deficient embryos at 25 hpf (Supplementary Fig. 5d ). Compared to the control group, Tg ( mpeg :GFP), a transgenic line of macrophages, also showed a reduction after nlrc3 knockdown at 30 hpf (Supplementary Fig. 5e ). These results reflected the role of nlrc3 signaling in primitive hematopoiesis. Since HSPCs originate from hemogenic endothelial cells in the dorsal aorta [33] , mutants or defects in blood vessel or artery genes may lead to hematopoietic defects. To explore this possibility, we examined the vascular endothelial-specific marker kdrl and the arterial-specific markers dlc at 26 hpf by WISH and found no notable vascular abnormalities in nlrc3 morphants or mutants (Supplementary Fig. 6a, b ). The same trend was observed in Tg ( kdrl :mCherry) at 28 hpf by confocal microscopy, and no alterations were observed between the different groups (Supplementary Fig. 6d ). Furthermore, the expressions of the endothelial and arterial markers dll4 , ephrinB2 , kdrl , and deltaC was not altered relative to the control group, as detected by qPCR (Supplementary Fig. 6c ). To further investigate whether the decrease in HSPCs in nlrc3 morphants was due to enhanced apoptosis in endothelial cells, we performed TUNEL in Tg ( fli1a :EGFP) embryos, which labels endothelial cells and were analyzed by confocal microscopy at 28hpf, the results indicated that loss of nlrc3 caused no increase in apoptotic endothelial cells within the DA (Supplementary Fig. 6e ), indicating that the defects in HSPCs in nlrc3- deficient embryos were not caused by apoptosis in endothelial cells. Taken together, these data imply that nlrc3 plays an imperative role in the definitive hematopoiesis of the zebrafish embryos. For the primitive wave, nlrc3 signaling was indispensable for the creation of neutrophils and macrophages. And this effect is not based on affecting the development of arterial vessels or causing apoptosis. As no previous studies have reported the involvement of nlrc3 in HSPC generation, we will investigate its underlying mechanism. Nlrc3 regulates HSPC emergence via activation of Notch signaling To determine the regulatory mechanism by which nlrc3 signaling regulates HSPCs, we sorted EGFP + cells in Tg ( fli1a : EGFP) zebrafish embryos at 28 hpf, which was the stage where EHT occurs in the VDA, and these EGFP + cells contained hemogenic endothelial cells (Fig. 4a ). Moreover, principal component analysis (PCA) indicated the high quality of our transcriptome profile data (Fig. 4b ). Fig. 4: RNA-seq demonstrates the regulatory mechanism underlying nlrc3 in HSPC emergence. a Schematic representation of RNA-seq analysis in this study. b Principal-component analysis (PCA) of six sequenced samples shown by the first three principal components (PC1–PC2). Control MO 1, blue; Control MO 2, light blue; Control MO 3, violet; nlrc3 MO 1, yellow; nlrc3 MO 2, green; nlrc3 MO 3, red; c Heatmap showing differential expression of hematologic-associated genes. The mark * indicates that there is a significant difference between the control group and morphant group with fold change >2 or fold change <0.5 and p -value < 0.05. (4) FDR < 0.05. d Representative statistically enriched biological process (BP), molecular function (MF) and cellular component (CC) associated genes of the upregulated and downregulated genes in nlrc3 morphant group compared with the control group. e Representative KEGG enrichment scatter plots of the signaling pathways in the nlrc3 morphant group compared with the control group. The plots were drawn based on the R version 4.1.3 and ggplot version 3.3.3. The statistical tests were one-sided and adjustments were made for multiple comparisons. f Expression of Notch genes in control embryos and nlrc3 morphants at 26 hpf by RNA-seq. Error bars, mean ± s.d., ns = 0.0554, 0.0645, 0.1207, * P = 0.0224, ** P = 0.0065, 0.0029, 0.0066, *** P = 0.0006, 0.0004, **** P < 0.0001, the exact p -values mentioned above are listed from left to right, by using two-tailed, unpaired Student’s t -test. n = 3 biological replicates. g Enrichment plot of the hematopoietic cell lineages between differentially regulated genes in the nlrc3 morphant group compared with the control group by GSEA (Gene Set Enrichment Analysis). P = 0.0465. h Enrichment plot of the Notch signaling pathway between differentially regulated genes in the nlrc3 morphant group compared with the control group by GSEA. P = 0.0003. GSEA of nlrc3 morphant versus control group transcriptional profiles using software GSEA (v4.1.0) and MSigDB, the statistical tests were one-sided and adjustments were made for multiple comparisons. Black bars indicate the individual genes, enrichment is in green. Normalized enrichment score = NES in ( g , h ). Source data are provided as a Source Data file. Full size image Based on the results of our RNA-Seq assays, a heatmap of differentially expressed genes (DEGs) showed hematologic-associated gene changes in the pathways related to nlrc3 in the morphant group (Fig. 4c ). As well as functional enrichment of common DEGs was performed, and GO analysis demonstrated changes in the categories of molecular function (MF), cellular component (CC) and biological process (BP) after knockdown nlrc3 (Fig. 4d ). To predict specific downstream pathways, KEGG pathway enrichment analysis was performed, and this analysis revealed that the upregulated DEGs were mainly involved in endocytosis and the MAPK signaling pathway, while the downregulated DEGs were mainly involved in multiple signaling pathways including TGF-β signaling, adherens junction, Wnt signaling, and Hedgehog signaling [34] , [35] . Among these pathways, Notch signaling was the most enriched in nlrc3 morphant (Fig. 4e ). Notch family genes were downregulated to varying degrees compared with the control groups, the nlrc3 knockdown groups showed different degrees of downregulation of notch-related genes, especially notch1a and hey1 specifically (Fig. 4f ). This trend was consistent with that of hematopoietic-related genes in Gene set enrichment analysis (GSEA) profiles (Fig. 4g, h ). These results strongly suggested that Notch signaling might be involved in nlrc3 -mediated regulation of HSPC emergence. To further explore this hypothesis, confocal microscopy images of the double-transgenic line Tg ( tp1 : EGFP/ kdrl :mCherry), which represented active Notch signaling, showed a reduced number of tp1 + kdrl + cells in the aortic floor at 30 hpf in nlrc3 -deficient embryos, and this phenotype was rescued by nlrc3 mRNA overexpression (Fig. 5a, b ). Similar trends were observed in transgenic Tg ( tp1 :EGFP) embryos at 48 hpf (Supplementary Fig. 7a ) [36] . Flow cytometry showed that the number of tp1 + cells was decreased when nlrc3 was inhibited, and this was restored by nlrc3 mRNA overexpression (Supplementary Fig. 7b, c ). Furthermore, in the RNA sequencing data, wnt16 showed a significant downregulation, which is considered a major regulator of Notch [37] , [38] . To further investigate the mechanism of nlrc3 regulation of Notch, we synthesized the mRNA of wnt16 for overexpression experiments. The results of WISH showed that the decreased expression of runx1 at 28hpf due to the loss of nlrc3 could be partially rescued by overexpression of wnt16 (Supplementary Fig. 8a, b ). The qPCR results also confirmed this phenotype (Supplementary Fig. 8c ). On the other hand, as significant regulators of the Notch signaling pathway and hematopoiesis during this specific developmental stage, we have identified genes in the RNA sequencing data that exhibit notable differences, including vegf and evi1 [35] , [39] , [40] . In order to further explore the regulatory mechanisms of nlrc3 , we synthesized their mRNA and performed overexpression experiments on nlrc3 mutants. However, the qPCR results indicate that the overexpression of vegfaa , vegfab , and evi1 cannot effectively rescue the downregulation of r unx1 and cmyb caused by nlrc3 knockout (Supplementary Fig. 9a–c ). The results above demonstrate that within the hematopoietic regulatory network governed by nlrc3 , many genes are perturbed, but it is the Notch signaling that serves as the downstream regulatory role of nlrc3 . Fig. 5: Nlrc3 regulates HSPC production via activating Notch signaling. a , b Confocal imaging showing Tg ( tp1 :EGFP; kdrl :mCherry) embryos at 30 hpf in the floor of the DA (white arrowheads) in control embryos, nlrc3 morphants, and nlrc3 morphants with overexpression of nlrc3 mRNA with quantification ( b ). * P = 0.0394, 0.0221, n = 8, 7, 7 embryos. c , d Confocal imaging showing the number of CD41 + cells at 72 hpf in the CHT (white arrowheads) of Tg ( CD41 :GFP) embryos in the control embryos, treatment group with Notch inhibitor DAPT, and treatment group with Notch inhibitor DAPT with overexpression of nlrc3 mRNA with quantification ( d ). ns = 0.6905, **** P < 0.0001, n = 17, 12, 11 embryos. e Expression of nlrc3 , runx1 , and NOTCH family genes in the control embryos, treatment group with the Notch inhibitor DAPT, and treatment group with the Notch inhibitor DAPT with overexpression of nlrc3 mRNA at 30 hpf by qPCR. ns > 0.9999, = 0.2217, 0.4466, * P = 0.0149, 0.0498, ** P = 0.0047, 0.0049, *** P = 0.0004, 0.0002, **** P < 0.0001. f hsp70 :Gal4; UAS :NICD-myc embryos injected with control MO and nlrc3 MO, WISH for runx1 was performed at 28 hpf. g , h Confocal imaging showing the number of runx1 + kdrl + cells in Tg ( runx1 :EGFP/ kdrl :mCherry) embryos at 32 hpf in the AGM (white arrowheads) in control embryos, nlrc3 morphants, and nlrc3 morphants with overexpression of hey1 mRNA with quantification ( h ). ** P = 0.0021, *** P = 0.0003, n = 11, 10, 10 embryos. i , j Confocal imaging showing the number of hematopoietic cells in Tg ( CD41 :GFP) embryos at 72 hpf in the CHT (white arrowheads) in control embryos, nlrc3 morphants, and nlrc3 morphants with overexpression of hey1 mRNA with quantification ( j ). * P = 0.0380, **** P < 0.0001, n = 18, 17, 16 embryos. k Expression of the HSPC marker runx1 in control embryos, nlrc3 mutants, treatment group with Notch inhibitor DAPT and treatment group with Notch inhibitor DAPT with overexpression of hey1 mRNA at 30 hpf by WISH. Error bars, mean ± s.d., * P < 0.05, ** P < 0.01, *** P < 0.001, **** P < 0.0001, the exact p -values mentioned above are listed from left to right, by using one-way ANOVA with –Sidak test in ( b , d , h , j ), two-way ANOVA with Tukey’s post hoc test in ( e ), n = 3 biological replicates in ( e ). For the box plots in ( b , d , h , j ), box limits extend from the 25th to 75th percentile, while the middle line represents the median. Whiskers extend to the largest value no further than 1.5 times the IQR from each box hinge. Scale bars, 100 μm in ( a , c , f , g , i , k ). Source data are provided as a Source Data file. Full size image To provide additional evidence from another perspective, we used the notch-specific inhibitor DAPT (N-[N-(3,5-difluorophenacetyl)-lalanyl]-S-phenylglycine t-butyl ester) to block the Notch signaling pathway to explore the relationship between nlrc3 and Notch signaling pathway. The WISH results showed that DAPT-treated embryos had decreased frequency of HSPC marker runx1 , but the overexpression of nlrc3 could not rescue these effects (Supplementary Fig. 8d ). Similarly, overexpression of nlrc3 could not rescue the levels of DAPT-treated CD41 + cells at 72 hpf (Fig. 5c, d ). Intriguingly, qPCR results showed that Notch family genes were decreased after DAPT treatment, but overexpression of nlrc3 mRNA barely rescued this drop, except for notch1a and hey1 at 30 hpf (Fig. 5e ), further indicating that nlrc3 acts in the upstream of Notch signaling. To test our hypothesis by rescue Notch, the double transgenic line Tg ( hsp70 : GAL4/ UAS : NICD), which contains the Notch intracellular domain (NICD), which can be triggered and enter the nucleus to play key biological roles during Notch activation, was used to ectopically activate Notch signaling by heat-shock induction after MO injection. In contrast to that of morphants, the overexpression of NICD effectively rescued the expression of runx1 + , as shown by WISH (Fig. 5f ). Furthermore, induction of NICD rescued the depletion of cmyb at 36 hpf and 48 hpf in nlrc3 morphants (Supplementary Fig. 7d ). Altogether, these data supported the hypothesis that nlrc3 activated the Notch signaling during hematopoiesis in zebrafish. Hey1 acts downstream of nlrc3 -Notch signaling in HSPC emergence To explore the mechanism by which nlrc3 induces Notch activation, qPCR was performed to analyze the expression of Notch ligands and target genes in nlrc3 -deficient embryos. Consistent with previous results and our RNA-seq analysis, the expression of notch1a decreased significantly and this decreasing trend could be rescued by overexpression of nlrc3 (Supplementary Fig. 8e ). Moreover, the expression of hey1 was significantly downregulated compared with other target genes (Supplementary Fig. 8f , Fig. 4f ), suggesting that nlrc3 plays a regulatory role through notch1a and hey1 . To prove whether hey1 was downstream of nlrc3 signaling, we synthesized hey1 mRNA for rescue experiments. To explore the effects of hey1 on the emergence and expansion stages of HSPCs, we used nlrc3 MOs with hey1 overexpression to determine the numbers of HSPCs at different time points, and we found that hey1 could rescue the decreased numbers of runx1 + kdrl + positive HSPCs at 32 hpf (Fig. 5g, h ) and CD41 + HSPCs in CHT at 72 hpf (Fig. 5i, j ). To validate the relationship between nlrc3 and hey1 at the mRNA level, we injected hey1 mRNA into nlrc3 mutants to verify its effect on multiple markers by qPCR. The results showed that overexpression of hey1 had no significant impact on the expression of nlrc3 but rescued the expression of HSPC markers ( runx1 , cmyb ) and hey1 -related genes edn1 and plxnd1 (Supplementary Fig. 9h ). Furthermore, WISH was performed after the morphant embryos were treated with the Notch signaling pathway inhibitor DAPT, and overexpression of hey1 mRNA also rescued the decreased expression of runx1 (Fig. 5k ). To examine the ability of HSPC differentiation, we measured the expression of myeloid, erythroid and lymphoid lineages respectively through Sudan Black [41] , gata1a , and rag1 at 96 hpf and found that hey1 could rescue these lineages under conditions of Notch inhibitor (Supplementary Fig. 9d–f ), indicating that the differentiation of HSPCs was repaired by this pathway. In summary, these findings suggest that hey1 was downstream of nlrc3 and that nlrc3 -Notch- hey1 axis triggers HSPC emergence and differentiation. Nlrc3 is downstream of the NF-kB signaling pathway in HSPC emergence Previous reports have revealed that the TLR4–MyD88–NF-kB signaling pathway is involved in regulating the production of HSPCs [1] , and correspondingly, nlrc3 was reported to attenuate Toll-like receptor signaling via modifying NF-kB with adults [7] . Therefore, we continued to explore the connection between NF-kB and nlrc3 during embryonic hematopoiesis. First, as previously described, RNA-seq analysis showed that the knockdown of nlrc3 did not affect the expression of the NF-kB pathway in GSEA (Supplementary Fig. 9i ). Specifically, after the knockdown of nlrc3 , NF-kB-related gene interleukin 1 beta ( il1b ), nfkbie and nfkbiz were upregulated, nfkbiab , nfkb2 and nfkbib were downregulated, nfkbiaa , nfkb1 , nfkbil1 and p65 were not statistically difference compared with the control group (Fig. 6a ). These results prompted us to examine whether nlrc3 might be regulated by NF-kB. Second, to explore the relationship between nlrc3 and NF-kB, IkBaa, the NF-kB inhibitory protein that normally binds to NF-kB and prevents the translocation of NF-kB to the nucleus, was knocked down by MO to increase the NF-kB activity. As shown by qPCR, expression of runx1 and NF-kB-related gene il1b was not significantly increased after overexpression of NF-kB in nlrc3 −/− mutants compared to the control group (Fig. 6b ). To verify this phenotype, we performed WISH and found that, compared to that in the control group, runx1 was activated due to knockdown of IkBaa. It was not increased in nlrc3 mutants even with the overexpression of NF-kB (Fig. 6c, d ). Besides, JSH-23, a target inhibitor of the nuclear translocation of NF-kB [42] , was administered to embryos with nlrc3 overexpression, and WISH analysis of runx1 and cmyb was performed at 36 hpf and 48 hpf, respectively. Both inhibitors-treated embryos showed significant reduction of runx1 or cmyb expression in the aortic floor, and nlrc3 mRNA could rescue the phenotypes (Fig. 6e, f , Supplementary Fig. 9g ). Similarly, to assess this trend during the expansion of HSPCs, these results were supported by the quantitation of CD41 + HSPCs at 72 hpf (Fig. 6g ). Third, to further evaluate whether NF-kB induced nlrc3 activation, qPCR analyses of embryos at 36 hpf showed that il1b , the NF-kB subunit p65 , was reduced after JSH-23 treated, but the overexpression of nlrc3 mRNA could not rescue this phenotype. Meanwhile, both expression levels of nlrc3 and hematopoiesis marker were increased following the enforced expression of nlrc3 (Fig. 6i ). In summary, these data confirmed that nlrc3 was downstream of NF–kB signaling pathway in transcription and that the NF-kB- nlrc3 -Notch- hey1 axis was both necessary and sufficient for HSPC emergence in zebrafish (Supplementary Fig. 9j ). Fig. 6: Nlrc3 is downstream of the NF-kB signaling pathway for regulating HSPC emergence. a Expression of NF-kB genes in control embryos and nlrc3 morphants at 26 hpf by RNA-seq. ns = 0.2176, 0.4498, 0.6039,0.1870, * P = 0.0224, 0.0311, ** P = 0.0022, 0.0018, 0.0083, *** P = 0.0002, **** P < 0.0001. b Expression of nlrc3 , runx1 , and the NF-kB target gene il1b in control embryos, nlrc3 mutants, nlrc3 mutants with ikbaa Mo, and treatment group with ikbaa Mo at 30 hpf by qPCR. ** P = 0.0041, 0.0053, *** P = 0.0001, **** P < 0.0001. c , d Expression of the HSPC marker runx1 in control embryos, ikbaa morphants, nlrc3 mutants, and nlrc3 mutants with ikbaa morphants at 28 hpf by WISH (black arrowheads) with quantification ( d ) ns = 0.3163, 0.9187, **** P < 0.0001, n = 12, 12, 14, 18 embryos. e , f Expression of the HSPC marker cmyb in control embryos, nlrc3 mutants, nlrc3 mutants with overexpression of nlrc3 mRNA, treatment group with NF-kB inhibitor JSH-23, and treatment group with NF-kB inhibitor JSH-23 and overexpression of nlrc3 mRNA at 48 hpf by WISH (black arrowheads) with quantification ( f ) **** P < 0.0001, n = 12, 21, 20, 11, 13 embryos. g , h Confocal imaging showing the number of CD41 + cells at 72 hpf in the CHT (white arrowheads) of Tg ( CD41 :GFP) embryos in the control embryos, treatment group with NF-kB inhibitor JSH-23, and treatment group with NF-kB inhibitor JSH-23 and overexpression of nlrc3 mRNA with quantification ( h ). * P = 0.0387, **** P < 0.0001, n = 17, 19, 16 embryos. i Expression of HSPC genes and NF-kB genes in control embryos, treatment group with NF-kB inhibitor JSH-23, and treatment group with NF-kB inhibitor JSH-23 with overexpression of nlrc3 mRNA at 30 hpf by qPCR. ns = 0.8444, 0.9785, * P = 0.0179, *** P = 0.0005, **** P < 0.0001. Error bars, mean ± s.d., * P < 0.05, ** P < 0.01, *** P < 0.001, **** P < 0.0001, the exact p -values mentioned above are listed from left to right, by using two-tailed, unpaired Student’s t -test in ( a ), one-way ANOVA with –Sidak test in ( d , f , h ), two-way ANOVA with Tukey’s post hoc test in ( b , i ), n = 3 biological replicates in ( a , b , i ). For the box plots in ( d , f , h ), box limits extend from the 25th to 75th percentile, while the middle line represents the median. Whiskers extend to the largest value no further than 1.5 times the IQR from each box hinge. Scale bars, 100 μm in ( c , e , g ). Source data are provided as a Source Data file. Full size image Nlrc3 signaling is conserved in the regulation of vertebrate hematopoiesis To further extend our findings in mammals, we utilized Nlrc3 knockout mice to explore whether Nlrc3 signaling was evolutionarily conserved in HSPCs emergence. We first verified the knockout efficiency at the Nucleic acid and protein levels (Supplementary Fig. 10a–c ). Then we found Nlrc3 −/− embryos showed developmental delays and Nlrc3 −/− FLs are smaller than wild-type at 14.5 days (E14.5) (Supplementary Fig. 10d ). Like the phenotype of our zebrafish model, we examined the AGM region of Nlrc3 −/− embryo to determine whether the production of HSPCs was changed (Fig. 7a ). Hematogenic endothelial cells (CD31 + CD41 − CD45 − TER119 − ) [43] from the embryonic AGM tissues at E10.5 were sorted and cultured in OP9 for 4 days (Fig. 7b ), and then, flow cytometry was performed to assess the proliferative capacity of these HSPCs. c-Kit + CD45 + hematopoietic cells were notably decreased in these Nlrc3 −/− embryos (Fig. 7c, d ). Correspondingly, to obtain more direct phenotypes, flow cytometry was also performed and showed that CD31 + Sca-1 + CD201 + hematopoietic stem cells were decreased in the AGM of Nlrc3 −/− embryos at E10.5 (Supplementary Fig. 10e–g ). Fig. 7: Nlrc3 signaling is conserved in the regulation of vertebrate hematopoiesis. a Schematic representation of AGM-derived hematopoietic endothelial (HE) cells. b Representative view of the hematopoietic cells (round) generated from 500 HE cells after co-culture with OP9 stromal cells for 4 days. c , d Flow cytometry results showing that after 4 days of OP9 co-culture, the number of c-Kit + CD45 + cells in Nlrc3 embryos decreased with quantification ( d ). *** P = 0.0001, n = 7, 6 embryos. e Schematic representation of fetal liver-derived cells performed in this study and flow cytometry results showing that the number of LT-HSC (Lin − c-Kit + Sca-1 + CD150 + CD48 − ) cells in Nlrc3 embryos decreased. f Percentage of LT-HSCs in 14.5 embryonic fetal liver of control embryos and Nlrc3 embryos. *** P = 0.0006, n = 5 embryos. g Quantification of LSK in 14.5 embryonic fetal liver of control embryos and Nlrc3 embryos. **** P < 0.0001, n = 6 embryos. h CFU-C assay of fetal liver showing that the number of CFU-mix, CFU-granulocyte-macrophage (CFU-GM), and CFU-erythroid (CFU-E) was decreased upon knock-down of Nlrc3 . * P = 0.0114, 0.0132, *** P = 0.0007, n = 3 biological replicates. i Schematic representation of bone marrow transplantation experiments performed in this study. j A total of 5 × 10 5 fetal liver-derived cells sorted from WT or Nlrc3 −/− mice were transplanted with 5 × 10 5 rescue cells into recipient mice. Peripheral blood (PB) analysis for the percentage of engrafted donor cells at the indicated number of weeks post-transplantation. * P = 0.0473, ** P = 0.0038, n = 4 biological replicates. k At 16 weeks post-transplantation, the PB of recipient mice transplanted with control or Nlrc3 −/− was analyzed for the percentage of donor-derived B, T, and myeloid cells. ** P = 0.0075, n = 3 biological replicates. l Flow cytometry results show the proportion of donor with control or Nlrc3 −/− in the BM of recipient mice at 16 weeks post-transplantation n = 5 biological replicates. m Quantification of the proportion of the donor-derived cell in BM. ** P = 0.0055, n = 4 biological replicates. n Expression of Nlrc3 , Runx1 , Il1b , and Notch-related genes in WT, Nlrc3 −/− whole FL at E14.5 by qPCR. ns = 0.8168, * P = 0.0137, 0.0205, 0.0107, ** P = 0.0078, 0.0039, 0.0063, **** P < 0.0001. Error bars, mean ± s.d., the exact p -values mentioned above are listed from left to right by using two-tailed, unpaired Student’s t -test in ( d , f , g , j , k , m , n ). Illustrations created with BioRender.com. Source data are provided as a Source Data file. Full size image To verify the phenotype of HSPCs in FL (Fig. 7e ), through flow analysis, we found that the proportion and absolute number of LT-HSC populations (Lin − c-Kit + Sca-1 + CD150 + CD48 − ) of FL cells from Nlrc3 −/− embryos were markedly decreased (Fig. 7f, g ). To test the function of Nlrc3 −/− FL-derived hematopoietic stem cells in vitro, by performing a colony-forming unit-cell (CFU-C) assay, we found compromised colony formation abilities of these FL HSCs from Nlrc3 −/− embryos (Fig. 7h ). To verify the functionality of Nlrc3 −/− embryonic HSCs in vivo, we performed BM transplantation experiments and observed a more than 3-fold reduction in the overall repopulation rate (Fig. 7i, j ). We also observed a myeloid lineage bias compared to that in the control group (Fig. 7k ). At 16 weeks post transplantation, the proportion of CD45.2 in the BM of recipient mice was reduced by more than 3 times compared to that of wild-type mice (Fig. 7l, m ). To verify the underlying mechanism of impaired HSC function in Nlrc3 −/− mice, we performed qPCR using mRNA from FL-derived LSK (Lin − c-Kit + Sca-1 + ) cells. The results showed that compared with the wild-type group, the Notch family-related genes were downregulated at the transcriptional level, and the expression of Hey1 was also decreased. This downward trend was consistent with that of Nlrc3 and the HSC marker Runx1 , while no significant changes were found in the NF-kB family gene Il1b (Fig. 7n ). Linking to the reported sequencing data during fetal EHT [28] , the expression of Notch1a and Hey1 significantly decreased in HSCs compared to HE, while the expression of Nlrc3 was increased (Supplementary Fig. 10h ). The above results further demonstrated that the NF-kB- Nlrc3 -Notch- Hey1 axis orchestrated development of embryonic HSCs was highly conserved in vertebrates (Supplementary Fig. 10j ). Inflammatory signaling is generally believed to be active in response to cell emergencies such as infection. Since inflammatory factors have an essential role in supporting HSPC proliferation and differentiation into mature immune cells in adults under stress-induced hematopoiesis [44] , [45] , the roles of PRRs and their regulatory mechanisms in early embryonic hematopoiesis warrant more attention. In this study, we demonstrated that a member of the NLR family, Nlrc3 , regulates HSPC emergence in vertebrates, which further highlights the roles of inflammasome signaling pathways in hematopoiesis and raises the question of whether their impacts are broader than previously thought. The current question is the role of NLRC3 in adult blood cells, such as myeloid cells. In the latest reports, Nlrc3 has been suggested to induce immune tolerance in monocytes and macrophages during polymicrobial sepsis [46] , In this context, the expression of Nlrc3 in myeloid cells becomes a reference point for monitoring such infections. Combining our analysis of NLRC3 expression in subpopulations of myeloid cells within the adult bone marrow, we observed enrichment in conjunction with inflammatory factors such as CSF2R and INFGR (Supplementary Fig. 10i ) [47] . On one hand, this indicates that Nlrc3 plays a crucial role from hematopoiesis to mature immune cells. On the other hand, it suggests that targeting NLRC3 in specific cells might be a promising candidate therapy. The contribution of Notch ligands, receptors, and target molecules to hematopoiesis has been extensively elucidated [13] , [14] , [48] . It is worth noting that this feature stems from the duality between arteriogenesis and hematopoiesis. Since arteries are thought to be the first niche for HSPCs, the differences in the association between arterial specification and definitive hematopoietic program underscore the intricacy of embryonic HSPCS development and the difficulty of recapitulating it in vitro. Our work not only clarifies the role of the crucial factors upstream of Notch but also expands our understanding of its downstream molecule hey1 , which has been recognized as a typical Notch downstream gene enriched in the cardiovascular system. Our findings promoted a more complete understanding of Notch and its roles in the regulation of hematopoiesis. Prior investigations have exhibited that Wnt16 engages in reciprocal interactions with Notch-related ligands, facilitating the specialization of hematopoietic stem cells [37] , [49] . Within this study, we observe that silencing of nlrc3 leads to a notable downregulation of wnt16 , while the closely linked Notch ligands deltaC and deltaD , along with notch3 , remain largely unaltered. This may potentially elucidate that the effects of nlrc3 signaling on wnt16 alteration persist until the EHT stage and beyond, encompassing later stages of hematopoietic development. Curiously, the conventional belief is that wnt16 modulation occurs prior to the emergence of HSPCs, yet it is intriguing that wnt9a [50] , another member of the Wnt family, which is conjectured to be related to the amplification of HSPCs, exhibits significant upregulation, albeit at a much later juncture around 32 hpf [51] . This outcome extends a broader scope for the exploration of the interplay between nlrc3 signaling and the Wnt family. What is more, the determination of arterial versus venous fate has been elucidated to hinge upon the Vegf–Notch pathway [52] , [53] . Interestingly, in the absence of nlrc3 signaling, varying degrees of downregulation are detected within the Vegf family. Nevertheless, notable downregulation of Vegf receptors flt4 and flk1 / kdrl remains absent, and the overexpression of vegfaa and vegfab mRNA fails to effectively rescue the defects in HSPCs. These two adverse outcomes might imply that the nlrc3 signal, acting as an upstream factor, influences Vegf even before the occurrence of HSPCs, whether it does directly participate in the initiation of HSPCs or not [54] . After all, our understanding remains limited regarding the intricate mechanisms through which Vegf orchestrates the initiation of HSPCs. The NF-kB family of transcription factors serve as regulators under stress conditions and are regarded as a regulator of the emergence of HSPCs that support hematopoietic homeostasis and regeneration [21] . Previous studies have revealed that Nlrc3 acts as a negative regulator of NF-KB [6] , [55] , through NF-KB, Myeloid-specific Nlrc3 deletion induced immunosuppression by improving macrophage glycolysis [46] . In this work, we established the mutual relationship between nlrc3 and NF-kB in vivo, showing that compared with adults, they have different regulatory relationships in embryonic stages. Different from negatively regulating NF-kB upstream, we propose that nlrc3 is regulated downstream of NF-kB. Consider the difference between embryonic and adult stages, understanding the evolutionary process of this role switch from embryos to adults requires in-depth research and tracking. Moreover, we delineated the network of the NF-kB pathway in the embryonic emergence of HSPCs, and we provided more perspectives deciphering the complete function of the NF-kB signaling pathway. Overall, by summarizing the results of the physiological and developmental roles in vivo and in vitro, we demonstrated that the NF-kB- Nlrc3 -Notch- Hey1 axis plays a key role in vertebrate HSPC emergence and differentiation. Our findings suggested that functional deficiency in the Nlrc3 mutant and morphant during HSPCs development under physiological conditions is of major importance since this investigation might be taken into consideration when recapitulation definitive hematopoiesis in vitro. The research complies with all relevant ethical regulations and was approved by the Laboratory Animal Center of Zhejiang University. The culture, differentiation, and sorting of embryonic stem cells (ESCs) in vitro The data of mESCs hematopoietic differentiation and RNA-seq derived from the publications [30] . The hematopoietic differentiation of hESCs was performed using STEMdiff Hematopoietic Kit (STEMCELL Technologies; 05310) following the instructions. Fluorescence-activated cell sorting (FACS) was performed according to the following two schemes, first based on the differentiation time point including day3, day6, day9 and day 12. Second, cells were sorted by the following markers: CD309-Percp/cy5.5 CD31-APC CD34-PE, CD43-APC and CD45- FITC (all kits Biolegend). The total RNA of these FACS-sorted cells was extracted into RNA by using Trizol reagent (Life Technologies; 15596026), and 1 μg RNA was reverse-transcribed into complementary DNA (cDNA) using HiScript II Q RT SuperMix for qPCR (+gDNA wiper) according to the manufacturer’s instructions (Vazyme; R223-01). Zebrafish and mouse strains All zebrafish strains were maintained in 28.5 °C system water in accordance with the relevant guidelines of the Laboratory Animal Center of Zhejiang University [17] . Male and female mice from 8 to 12 weeks old were used for all studies. The mice used included C57 wild-type CD45.2, Nlrc3 knockout mice with CD45.2, and CD45.1 mice. All mice were cultured in a suitable temperature and humidity environment and fed with sufficient water and food (25 °C, suitable humidity (typically 50%), dark/light cycle for 12 h); the morning in which a vaginal plug was observed in the female was defined as embryonic day 0.5 (E0.5). All procedures of the animal experiments were reviewed and approved by the Institutional Animal Care and Use Committee of the Laboratory Animal Center, Zhejiang University (Reference No. : ZJU20230065). Injection of morpholino Splice Modifying morpholinos (MOs) used in our study were ordered from Gene Tools. The MOs were diluted in diethyl pyrocarbonate-treated water at a concentration of 0.2 mM (Standard-MO) and 2 mM ( Nlrc3 MO) with phenol red solution, and 1 nl indicated MO was injected into one-cell stage embryos. 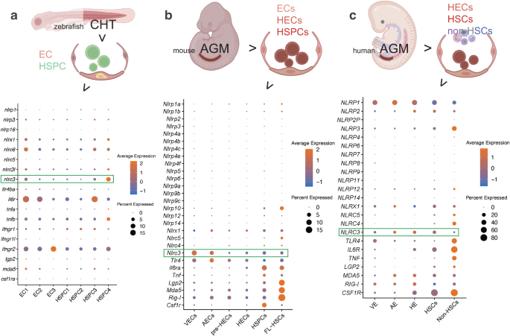Fig. 1:NLRC3is highly expressed during vertebrates HSPC development. aSchematic paradigm of zebrafish caudal hematopoietic tissue (CHT) tissue for single-cell RNA-seq (scRNA-seq) profiling. Bubble plot of scRNA-Seq data demonstrating the expression of nucleotide-binding domain leucine-rich repeat (NLR) family members, includingNlrc3and related inflammatory genes in the clusters of endothelial cells (ECs) and Hematopoietic stem and progenitor cells (HSPCs).bSchematic paradigm of mouse embryonic Aorta Gonad Mesonephros (AGM) for scRNA-seq profiling. Bubble plot of scRNA-Seq data demonstrating the expression of NLR family members, includingNlrc3and related inflammatory genes in the clusters of venous endothelial cells (VECs), arterial endothelial cells (AECs), pre-hemogenic endothelial cells (pre-HECs), hemogenic endothelial cells (HECs), HSPCs, fetal liver (FL)-derived HSPCs.cSchematic paradigm of human embryonic AGM for scRNA-seq profiling. Bubble plot of scRNA-Seq data demonstrating the expression of NLR family members, includingNLRC3and inflammatory genes in the clusters of venous endothelium (VE), arterial endothelium (AE), hemogenic endothelium (HE), HSPCs and Non-HSCs. Illustrations created with BioRender.com. Source data are provided as a Source Data file. The sequences of MOs used in this study are listed in Supplementary Table 1 . Generation of zebrafish knockout lines using CRISPR/Cas9 In brief, a target site ( GGTCTACTGTCGCCCACAGC TGG) in exon 1 of the nlrc3 gene was chosen, and the guide RNA (gRNA) template was amplified from the pMD-gata5-gRNA scaffold vector. In vitro transcription was performed using 1 μg of template DNA and T7 RNA polymerase. Zebrafish codon-optimized Cas9 plasmid was linearized with Xba I, and Cas9-capped mRNA was transcribed using the T7 High Yield RNA Transcription Kit (Vazyme; TR101-01). The size and quality of the capped mRNA and gRNA were confirmed by electrophoresis through a 2% (w/v) agarose gel. Subsequently, 100 pg of gRNA and 400 pg of Cas9 mRNA (New England Biolabs; M0646T) for microinjection into one-cell stage embryos. The following primer pairs and the restriction enzyme Bst XI were used to assess the efficiency of genetic disruption: forward5’-ACTTTGGGTCGTCTTGCTTTTTA-3’, reverse5’-AACAAATAGGCGAGAACAGCACA-3’. F0 embryos with the highest editing efficiency were raised. Heterozygous F1 fish were identified using DNA sequencing of the offspring of F0 fish outcrosses. The mutant and wild-type animals were obtained from heterozygous crosses. Confocal microscopy Transgenic embryos including Tg( lcr :EGFP), Tg( gata1a :DsRed), Tg( mpx :EGFP), Tg( lyz :DsRed), Tg( mpeg :EGFP), Tg( lck :EGFP), Tg( fli1a :EGFP), Tg( tp1 :EGFP), Tg( CD41 :GFP) and Tg( runx1 :EGFP; kdrl :mCherry), Tg( cmyb :GFP; kdrl :mCherry) double-transgenic embryos were anesthetized and mounted on dishes with 0.8% low-melting agarose. Confocal images of the Z sections of the head, DA or CHT region were photographed by an FV1000 microscope (Olympus) to visualize HSPCs and lineages at each time point. The analysis of the images was carried out by Olympus confocal software Image J. Whole-mount in situ hybridization Whole-mount in situ hybridization (WISH) was performed as described [56] with slight modifications. Probes for nlrc3 , runx1 , cmyb , gata1a , rag1 , mpx , foxn1 , kdrl , dlc , l-plastin , and mfap4 transcripts were generated using a DIG RNA Labeling Kit (Roche; 11175025910) from relevant linearized plasmids. Embryos were observed and photographed by a Nikon SMZ18 stereo microscope. Sudan black staining and o -dianisidine staining Sudan Black staining was used to detect the granules of the granulocytes [57] . Fixed larvae were rinsed in PBT (phosphate-buffered saline, PBS with 0.1% Tween-20; Sigma-Aldrich) twice for 5 min and incubated in 1 mL Sudan Black (Sigma-Aldrich) for 20 min. To stop the staining process, the embryos were washed two times in 70% ethanol for 15 min and passage into 30% ethanol and imaged using a Nikon SMZ18 stereo microscope. o -Dianisidine staining was used to check the hemoglobin; a brown color indicated the presence of hemoglobin in zebrafish embryos. Before staining, a stock solution of 100 mg o-dianisidine dissolved in 70 mL ethanol was prepared at 4 °C in the dark. For staining, live embryos were exposed to an o-dianisidine working solution consisting of 2 mL o-dianisidine stock solution, 0.1 m sodium acetate (pH 4.5), and 0.65% H2O2 in a small glass bottle for 3–5 min at room temperature. To stop the staining process, the embryos were washed two times in PBS and were imaged using a Nikon SMZ18 stereo microscope. Quantitative real-time PCR analysis Total RNA was isolated from FACS-sorted cells or each time point dissected regions that included caudal hematopoietic tissue (CHT) or heads of zebrafish by using Trizol and 1 μg RNA was reverse-transcribed into complementary DNA (cDNA) using HiScript II Q RT SuperMix for qPCR (Vazyme; R222-01) according to the manufacturer’s protocol. Quantitative PCR (qPCR) was performed on a Bio-Rad CFX96 system using ChamQ Universal SYBR qPCR Master Mix (Vazyme; Q711-02/03) and samples were run in duplicate or triplicate with R3 biological replicate pools/condition. Each sample was performed in triplicate and all results were normalized to the expression of Actin. Data are represented as mean 6 standard deviations (SD), and significance was determined by two-tailed Student’s t -tests between control and experimental groups. 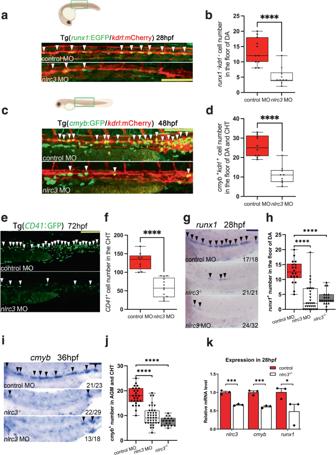Fig. 2:Nlrc3signaling is indispensable for HSPC production in zebrafish. a,bConfocal imaging showing the number of hemogenic endothelium and emerging HSPCs inrunx1+kdrl+cells from Tg (runx1:EGFP/kdrl:mCherry) embryos at 28 hpf in the AGM (white arrowheads) in control embryos andnlrc3morphants with quantification (b). ****P< 0.0001,n= 11, 10 embryos.c,dConfocal imaging showing the number ofcmyb+kdrl+cells in Tg (cmyb:EGFP/kdrl:mCherry) embryos at 48 hpf in the AGM (white arrowheads) in control embryos andnlrc3morphants with quantification (d). ****P< 0.0001,n= 10, 9 embryos.e,fConfocal imaging showing the number of HSPCs in Tg (CD41:GFP) embryos at 72 hpf in the CHT (white arrowheads) in control embryos andnlrc3morphants with quantification (f). ****P< 0.0001,n= 9, 13 embryos.g,hExpression of the HSPC markerrunx1innlrc3morphants and mutants in the AGM region at 28 hpf by whole mount in situ hybridization (WISH) (black arrowheads) with quantification (h) ****P< 0.0001,n= 18, 32, 21 embryos.i,jExpression of the HSPC markercmybinnlrc3morphants and mutants in the region of AGM and CHT at 36 hpf by WISH (black arrowheads) with quantification (j) ****P< 0.0001,n= 25, 37, 18 embryos.kExpression ofnlrc3and the HSPC genesrunx1,cmybin control embryos andnlrc3morphants at 28 hpf by qPCR. *P= 0.0462, ***P= 0.0006, 0.0010,n= 3 biological replicates. Error bars, mean ± s.d., ****P< 0.0001, by using two-tailed, unpaired Student’st-test in (b,d,f,k), one-way ANOVA – Sidak test in (h,j). For the box plots in (b,d,f,h,j), box limits extend from the 25th to 75th percentile, while the middle line represents the median. Whiskers extend to the largest value no further than 1.5 times the inter-quartile range (IQR) from each box hinge. Scale bars, 100 μm in (a,c,e,g,i). Illustrations created with BioRender.com. Source data are provided as a Source Data file. The PCR primers used are listed in Supplementary Table 2 . mRNA synthesis and injections For messenger RNA (mRNA) synthesis, total RNA was extracted from zebrafish wild-type embryos and reverse transcribed into cDNA. Specific primers were utilized to amplify the opening reading frame of nlrc3 , hey1 , wnt16 , gata2b , vegfaa , vegfab , evil . The PCR product was cloned into the pCS2+ plasmid and validated by bidirectional sequencing. The recombined pCS2+- nlrc3 , vegfaa , vegfab , wnt16 , evil plasmid was linearized by NotI and pCS2+- hey1 , gata2b , plasmid was linearized by BamHI and purified by FastPure Gel DNA Extraction Mini Kit (Vazyme; DC301-01). All of these capped full-length zebrafish mRNAs were generated by using SP6 mMESSAGE mMACHINE mRNA transcription synthesis kit (Invitrogen; AM1344) and cleaned up using RNA clean Kit (TIANGEN; DP412) according to the manufacturer’s instructions. Then, 100 pg purified nlrc3 and hey1 mRNA was injected into one-cell stage embryos alone or in combination with specific MOs. TUNEL assay and staining The TUNEL assay was performed using the fluorescein-based In Situ Cell Death Detection Kit (Roche; 12156792910) in accordance with the manufacturer’s instructions. Manually dechorionated Tg( fli1a :EGFP) transgenic embryos were fixed in 4% PFA at 4 °C overnight, washed three times with PBST and dehydrated in 100% methanol at −20 °C for more than 2 h. After gradual rehydration, embryos were washed with PBST three times, followed by proteinase K and acetone treatment. After washing 3 times with PBST, the permeabilized embryos were incubated in a mixture containing labeling solution and enzyme solution at a ratio of 9:1 at 4 °C overnight. Finally, the embryos were washed three times with PBST and then were captured by confocal microscopy. Note that anti-GFP (Invitrogen; A-11120) and Alexa Fluor 488-conjugated goat anti-mouse (Invitrogen; A-10680) antibodies were used as the primary and secondary antibodies, respectively. RNA-seq and bioinformatics analysis RNA-seq analysis was performed by LC-Bio Technology Co., Ltd [4] . Total RNA was extracted from sorted EGFP + cells in Tg( fli1a : EGFP) zebrafish embryos by using TRIzol Reagent following the manufacturer’s instructions. cDNA libraries were constructed by SuperScript™ II Reverse Transcriptase (Invitrogen; 18064014), and 150-bp single-end reads were generated on an Illumina HiSeq 6000 platform following the vendor’s recommended protocol. After removing the low-quality bases and undetermined bases by Cutadapt software (version: cutadapt-1.9), we used HISAT2 software (version: hisat2-2.0.4) to map reads to the genome (Ensembl Danio reio v96). The mapped reads of each sample were assembled using StringTie (version: stringtie-1.3.4d.) with default parameters. Then, all transcriptomes from all samples were merged to reconstruct a comprehensive transcriptome by using gffcompare software (version: gffcompare-0.9.8.). After the final transcriptome was generated, StringTie and ballgown were used to estimate the expression levels of all transcripts and perform expression level for mRNAs by calculating FPKM. The differentially expressed mRNAs were selected with fold change >2 or fold change <0.5 and p -value < 0.05 by R package edgeR ( http://www.r-project.org/ ) or DESeq2, and then analysis GO enrichment and KEGG enrichment to the differentially expressed mRNAs. Chemical treatment Zebrafish embryos were exposed to chemicals from the 10-somite stage to 24 hpf or 36 hpf. For evaluation of HSPCs development, exposure ranged until fixation and was subjected to WISH for runx1 , cmyb and rag1 . Siblings treated with 0.1% DMSO in Hotter buffer were taken as controls. Embryos with 100 µM DAPT (Calbiochem; 565770) [17] or 300 mM JSH-23 (Selleck; S7351) [1] were treated as treatment groups. Heat-shock treatment For induction of hsp70l : Gal4-driven NICD overexpression, embryos were placed to 37 °C heat shock at 18 hpf for 50 min. The embryos were then kept at 28 °C until each time point when they were fixed and processed for WISH. Flow cytometry analysis and cell sorting Cells derived from in vitro human ESC hematopoietic differentiation or tissue of mouse were harvested and suspended in PBS with 2% fetal bovine serum (FBS). Before antibody incubation, cells were blocked with an anti-CD16/32 antibody (eBioscience). Fluorescence-activated cell sorting (FACS) was based on the following markers: TER119- APC/Cyanine7, CD31-APC, CD45-FITC, CD41-PE/cy7, c-Kit-PE/cy5. Sca-1-APC, CD150-FITC, CD48-PE, CD201-FITC, CD45.1-AF-700 (all kits Biolegend). A different lineage cocktail (Lin) was used, including CD3, CD4, CD8, Gr1, B220, IgM and Ter119 [58] , [59] . 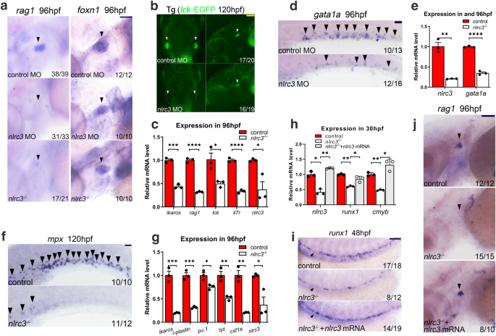Fig. 3:Nlrc3signaling is imperative for HSPC differentiation in zebrafish. aExpression of the lymphoid markerrag1innlrc3morphants and mutants and the thymic epithelial cell markerfoxn1in the thymus of control embryos,nlrc3morphants, and mutants at 96 hpf (black arrowheads).bSnapshot oflck+cells in Tg (lck:EGFP) embryos in the thymus of control embryos andnlrc3morphants at 5 dpf (white arrowheads).cExpression ofnlrc3and the lymphoid genesikaros,rag1,lck, andil7rin control embryos andnlrc3morphants at 96 hpf by qPCR. *P= 0.0229, 0.0197, ***P= 0.0009.dExpression of the erythroid markergata1ain control embryos andnlrc3morphants by WISH at 96 hpf (black arrowheads).eExpression ofnlrc3and the erythroid genegata1ain control embryos andnlrc3morphants at 96 hpf by qPCR. **P= 0.0011.fExpression of the myeloid markermpxin control andnlrc3morphants by WISH at 120 hpf (black arrowheads).gExpression ofnlrc3and the myeloid geneikaros, l-plastin, pu.1, lyz, andcsf1ain control embryos andnlrc3mutants at 96 hpf by qPCR. *P= 0.0178, 0.0197, **P= 0.0049, 0.0011, ***P= 0.0007, 0.0003.hExpression ofnlrc3and the HSPC genesrunx1andcmybin control,nlrc3morphants, andnlrc3morphants with overexpression ofnlrc3mRNA at 30 hpf by qPCR. *P= 0.0286, 0.0272, 0.0158, **P= 0.0040, 0.0047, 0.0068.iExpression of the HSPC markerrunx1in control embryos,nlrc3morphants, andnlrc3morphants with overexpression ofnlrc3mRNA at 48 hpf by WISH (black arrowheads).jExpression of the lymphoid markerrag1in control embryos,nlrc3morphants, andnlrc3morphants with overexpression ofnlrc3mRNA at 96 hpf by WISH (black arrowheads). Error bars, mean ± s.d., *P< 0.05, **P< 0.01, ***P< 0.001, ****P< 0.0001, the exactp-values mentioned above are listed from left to right, by using two-tailed, unpaired Student’st-test in (c,e,g). Two-way ANOVA with Tukey’s post hoc test in (h).n= 3 biological replicates. Scale bars, 100 μm in (a,b,d,f,i,j). Illustrations created with BioRender.com. Source data are provided as a Source Data file. DAPI was included to omit dead cells. Cells were stained in PBS/2% FBS for 30 min at room temperature and sorted out using BD AriaII (BD Biosciences). As for zebrafish, embryos were manually dechorionated with pronase, anesthetized in tricaine, dissociated with liberase, and triturated using a P1000 pipette. The resulting single-cell suspension was filtered with a 40-μm cell strainer and resuspended in PBS. Flow cytometric acquisitions or FACS were performed on BD Fortessa and BD AriaII (BD Biosciences), respectively. Graphs were prepared in FlowJo. Mouse embryo dissociation and FACS E10.5 AGMs (36–40 somite pairs) or E14.5 fetal livers were isolated from 6- to 8-week-old pregnant female mice, the tissues were isolated under a dissecting microscope, and cell suspensions were prepared in PBS containing 2% FBS by repeatedly flushing through needles ranging from 18- to 27-gauge. The cells were then passed through a nylon mesh with a pore size of 70 μm, and red blood cells were lysed using RBC lysis buffer (eBioscience; 00-4333-57). After dissociated by collagenase from WT and Nlrc3 −/− embryos, at least 500 CD31 + CD41 − CD45 − TER119 − cells from E10.5 AGMs were sorted by FACS and cultured on mouse OP9 stromal cells and supplemented with hematopoietic cytokines (50 ng/mL stem cell factor, 50 ng/mL IL3, 20 ng/mL FLT3 ligand). After being cultured for 4 days, semi-adherent cells were carefully harvested for flow cytometry. For staining LT-HSCs, the E14.5 fetal liver cells were first incubated with Fc-Block followed by biotin-conjugated lineage marker antibodies (PE/cy5-conjugated c-Kit, APC-conjugated Sca-1, FITC-conjugated CD150, PE-conjugated CD48). All antibodies were purchased from eBioscience or BioLegend. FACS data were analyzed using FlowJo software. In vitro methylcellulose colony-forming assays Fetal liver suspensions were prepared in Iscove’s Modified Dulbecco’s Medium (IMDM) supplemented with 2% FBS, and red blood cells were lysed using an RBC lysis buffer. A total of 3 × 10 4 FL cells were seeded in MethoCult M3434 (STEMCELL Technologies, 03434) containing recombinant mouse stem cell factor (SCF; 50 ng mL −1 ), recombinant mouse IL-3 (10 ng mL −1 ), recombinant human IL-6 (10 ng mL −1 ), and erythropoietin (U mL −1 ). All assays were performed in triplicate in a 35-mm culture dish incubated at 37 °C in humidified air containing 5% CO 2 for 12 days. The colonies were counted based on standard morphological criteria. BFU-E (burst-forming unit-erythroid), CFU-GM (colony-forming unit-granulocyte/macrophage), and CFU-GEMM (colony-forming unit-granulocyte/erythroid/macrophage/megakaryocyte) were classified and enumerated based on morphological recognition. Transplantation experiments Competitive reconstitution assays were performed as previously reported [6] , [7] . Eight-week-old CD45.1 mousse was lethally irradiated to a split dose of 9 Gy X-ray. Embryo equivalent cells from WT (CD45.2) or Nlrc3 −/− (CD45.2) fetal liver were mixed in a 1:1 and 1:4 ratio with 1 × 10 6 CD45.1 bone marrow cells and injected into recipient mice into the tail vein. 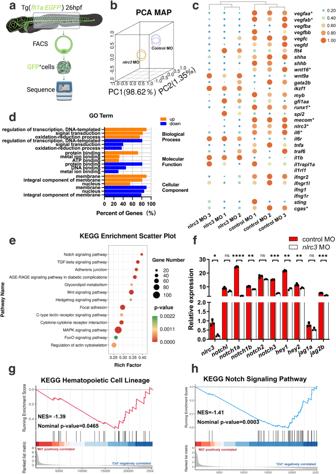Fig. 4: RNA-seq demonstrates the regulatory mechanism underlyingnlrc3in HSPC emergence. aSchematic representation of RNA-seq analysis in this study.bPrincipal-component analysis (PCA) of six sequenced samples shown by the first three principal components (PC1–PC2). Control MO 1, blue; Control MO 2, light blue; Control MO 3, violet;nlrc3MO 1, yellow;nlrc3MO 2, green;nlrc3MO 3, red;cHeatmap showing differential expression of hematologic-associated genes. The mark * indicates that there is a significant difference between the control group and morphant group with fold change >2 or fold change <0.5 andp-value < 0.05. (4) FDR < 0.05.dRepresentative statistically enriched biological process (BP), molecular function (MF) and cellular component (CC) associated genes of the upregulated and downregulated genes innlrc3morphant group compared with the control group.eRepresentative KEGG enrichment scatter plots of the signaling pathways in thenlrc3morphant group compared with the control group. The plots were drawn based on the R version 4.1.3 and ggplot version 3.3.3. The statistical tests were one-sided and adjustments were made for multiple comparisons.fExpression of Notch genes in control embryos andnlrc3morphants at 26 hpf by RNA-seq. Error bars, mean ± s.d., ns = 0.0554, 0.0645, 0.1207, *P= 0.0224, **P= 0.0065, 0.0029, 0.0066, ***P= 0.0006, 0.0004, ****P< 0.0001, the exactp-values mentioned above are listed from left to right, by using two-tailed, unpaired Student’st-test.n= 3 biological replicates.gEnrichment plot of the hematopoietic cell lineages between differentially regulated genes in thenlrc3morphant group compared with the control group by GSEA (Gene Set Enrichment Analysis).P= 0.0465.hEnrichment plot of the Notch signaling pathway between differentially regulated genes in thenlrc3morphant group compared with the control group by GSEA.P= 0.0003. GSEA ofnlrc3morphant versus control group transcriptional profiles using software GSEA (v4.1.0) and MSigDB, the statistical tests were one-sided and adjustments were made for multiple comparisons. Black bars indicate the individual genes, enrichment is in green. Normalized enrichment score = NES in (g,h). Source data are provided as a Source Data file. Then peripheral blood was collected from the tail and stained for CD45.1 and CD45.2 antibody at indicated time points. At 16 weeks after transplantation, bone marrow cells and peripheral blood were obtained and detected by flow cytometry. For competitive transplantation, 8-week-old CD45.1 + mice were lethally irradiated to a split dose of 9 Gy X-ray. Nucleated donor cells (CD45.2 + ) obtained from E14.5 WT and Nlrc3 −/− fetal livers were mixed with freshly isolated bone marrow nucleated cells (CD45.1 + ) in a 1:1 and 1:4 ratio, and the mixture was injected into the caudal vein of CD45.1 + mice. Then peripheral blood was collected from the tail and stained for CD45.1-PE and CD45.2-APC antibody at indicated time points from the recipients 4, 8, and 12 weeks for flow cytometric analysis. At 16 weeks after transplantation, bone marrow cells and peripheral blood were obtained and detected by flow cytometry. Statistical analysis All statistical analyses were generated using GraphPad Prism software (Prism 9). Values are shown as the mean ± standard deviation (SD). 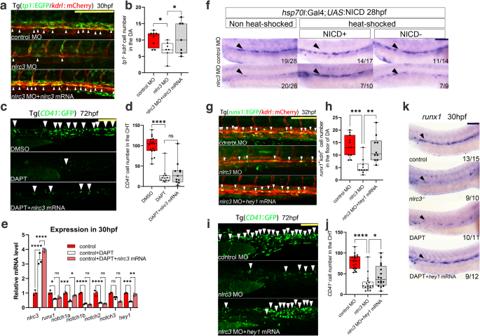Fig. 5:Nlrc3regulates HSPC production via activating Notch signaling. a,bConfocal imaging showing Tg (tp1:EGFP;kdrl:mCherry) embryos at 30 hpf in the floor of the DA (white arrowheads) in control embryos,nlrc3morphants, andnlrc3morphants with overexpression ofnlrc3mRNA with quantification (b). *P= 0.0394, 0.0221,n= 8, 7, 7 embryos.c,dConfocal imaging showing the number ofCD41+cells at 72 hpf in the CHT (white arrowheads) of Tg (CD41:GFP) embryos in the control embryos, treatment group with Notch inhibitor DAPT, and treatment group with Notch inhibitor DAPT with overexpression ofnlrc3mRNA with quantification (d). ns = 0.6905, ****P< 0.0001,n= 17, 12, 11 embryos.eExpression ofnlrc3,runx1, and NOTCH family genes in the control embryos, treatment group with the Notch inhibitor DAPT, and treatment group with the Notch inhibitor DAPT with overexpression ofnlrc3mRNA at 30 hpf by qPCR. ns > 0.9999, = 0.2217, 0.4466, *P= 0.0149, 0.0498, **P= 0.0047, 0.0049, ***P= 0.0004, 0.0002, ****P< 0.0001.fhsp70:Gal4;UAS:NICD-myc embryos injected with control MO andnlrc3MO, WISH forrunx1was performed at 28 hpf.g,hConfocal imaging showing the number ofrunx1+kdrl+cells in Tg (runx1:EGFP/kdrl:mCherry) embryos at 32 hpf in the AGM (white arrowheads) in control embryos,nlrc3morphants, andnlrc3morphants with overexpression ofhey1mRNA with quantification (h). **P= 0.0021, ***P= 0.0003,n= 11, 10, 10 embryos.i,jConfocal imaging showing the number of hematopoietic cells in Tg (CD41:GFP) embryos at 72 hpf in the CHT (white arrowheads) in control embryos,nlrc3morphants, andnlrc3morphants with overexpression ofhey1mRNA with quantification (j). *P= 0.0380, ****P< 0.0001,n= 18, 17, 16 embryos.kExpression of the HSPC markerrunx1in control embryos,nlrc3mutants, treatment group with Notch inhibitor DAPT and treatment group with Notch inhibitor DAPT with overexpression ofhey1mRNA at 30 hpf by WISH. Error bars, mean ± s.d., *P< 0.05, **P< 0.01, ***P< 0.001, ****P< 0.0001, the exactp-values mentioned above are listed from left to right, by using one-way ANOVA with –Sidak test in (b,d,h,j), two-way ANOVA with Tukey’s post hoc test in (e),n= 3 biological replicates in (e). For the box plots in (b,d,h,j), box limits extend from the 25th to 75th percentile, while the middle line represents the median. Whiskers extend to the largest value no further than 1.5 times the IQR from each box hinge. Scale bars, 100 μm in (a,c,f,g,i,k). Source data are provided as a Source Data file. The sample size for each statistical analysis is provided in the figure legends. Where indicated, two-tailed, unpaired Student’s t -test was used for comparisons between two groups, whereas one-way ANOVA was used for more than two groups’ comparisons. The log-rank test was used to analyze the survival curves. * P < 0.05 was considered statistically significant, ** P < 0.01, *** P < 0.001, **** P < 0.0001; n.s., not significant. 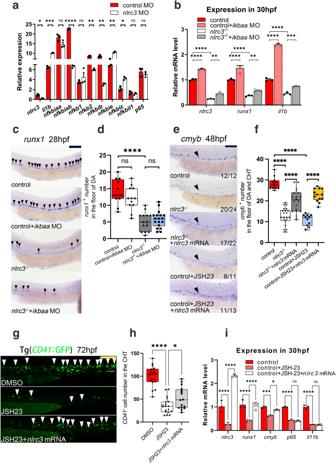Fig. 6:Nlrc3is downstream of the NF-kB signaling pathway for regulating HSPC emergence. aExpression of NF-kB genes in control embryos andnlrc3morphants at 26 hpf by RNA-seq. ns = 0.2176, 0.4498, 0.6039,0.1870, *P= 0.0224, 0.0311, **P= 0.0022, 0.0018, 0.0083, ***P= 0.0002, ****P< 0.0001.bExpression ofnlrc3,runx1, and the NF-kB target geneil1bin control embryos,nlrc3mutants,nlrc3mutants withikbaaMo, and treatment group withikbaaMo at 30 hpf by qPCR. **P= 0.0041, 0.0053, ***P= 0.0001, ****P< 0.0001.c,dExpression of the HSPC markerrunx1in control embryos,ikbaamorphants,nlrc3mutants, andnlrc3mutants withikbaamorphants at 28 hpf by WISH (black arrowheads) with quantification (d) ns = 0.3163, 0.9187, ****P< 0.0001,n= 12, 12, 14, 18 embryos.e,fExpression of the HSPC markercmybin control embryos,nlrc3mutants,nlrc3mutants with overexpression ofnlrc3mRNA, treatment group with NF-kB inhibitor JSH-23, and treatment group with NF-kB inhibitor JSH-23 and overexpression ofnlrc3mRNA at 48 hpf by WISH (black arrowheads) with quantification (f) ****P< 0.0001,n= 12, 21, 20, 11, 13 embryos.g,hConfocal imaging showing the number ofCD41+cells at 72 hpf in the CHT (white arrowheads) of Tg (CD41:GFP) embryos in the control embryos, treatment group with NF-kB inhibitor JSH-23, and treatment group with NF-kB inhibitor JSH-23 and overexpression ofnlrc3mRNA with quantification (h). *P= 0.0387, ****P< 0.0001,n= 17, 19, 16 embryos.iExpression of HSPC genes and NF-kB genes in control embryos, treatment group with NF-kB inhibitor JSH-23, and treatment group with NF-kB inhibitor JSH-23 with overexpression ofnlrc3mRNA at 30 hpf by qPCR. ns = 0.8444, 0.9785, *P= 0.0179, ***P= 0.0005, ****P< 0.0001. Error bars, mean ± s.d., *P< 0.05, **P< 0.01, ***P< 0.001, ****P< 0.0001, the exactp-values mentioned above are listed from left to right, by using two-tailed, unpaired Student’st-test in (a), one-way ANOVA with –Sidak test in (d,f,h), two-way ANOVA with Tukey’s post hoc test in (b,i),n= 3 biological replicates in (a,b,i). For the box plots in (d,f,h), box limits extend from the 25th to 75th percentile, while the middle line represents the median. Whiskers extend to the largest value no further than 1.5 times the IQR from each box hinge. Scale bars, 100 μm in (c,e,g). Source data are provided as a Source Data file. 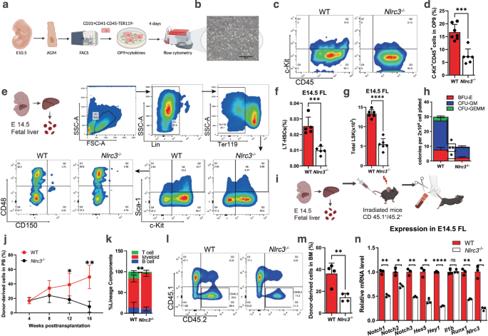Fig. 7:Nlrc3signaling is conserved in the regulation of vertebrate hematopoiesis. aSchematic representation of AGM-derived hematopoietic endothelial (HE) cells.bRepresentative view of the hematopoietic cells (round) generated from 500 HE cells after co-culture with OP9 stromal cells for 4 days.c,dFlow cytometry results showing that after 4 days of OP9 co-culture, the number of c-Kit+CD45+cells inNlrc3embryos decreased with quantification (d). ***P= 0.0001,n= 7, 6 embryos.eSchematic representation of fetal liver-derived cells performed in this study and flow cytometry results showing that the number of LT-HSC (Lin−c-Kit+Sca-1+CD150+CD48−) cells inNlrc3embryos decreased.fPercentage of LT-HSCs in 14.5 embryonic fetal liver of control embryos andNlrc3embryos. ***P= 0.0006,n= 5 embryos.gQuantification of LSK in 14.5 embryonic fetal liver of control embryos andNlrc3embryos. ****P< 0.0001,n= 6 embryos.hCFU-C assay of fetal liver showing that the number of CFU-mix, CFU-granulocyte-macrophage (CFU-GM), and CFU-erythroid (CFU-E) was decreased upon knock-down ofNlrc3. *P= 0.0114, 0.0132, ***P= 0.0007,n= 3 biological replicates.iSchematic representation of bone marrow transplantation experiments performed in this study.jA total of 5 × 105fetal liver-derived cells sorted from WT orNlrc3−/−mice were transplanted with 5 × 105rescue cells into recipient mice. Peripheral blood (PB) analysis for the percentage of engrafted donor cells at the indicated number of weeks post-transplantation. *P= 0.0473, **P= 0.0038,n= 4 biological replicates.kAt 16 weeks post-transplantation, the PB of recipient mice transplanted with control orNlrc3−/−was analyzed for the percentage of donor-derived B, T, and myeloid cells. **P= 0.0075,n= 3 biological replicates.lFlow cytometry results show the proportion of donor with control orNlrc3−/−in the BM of recipient mice at 16 weeks post-transplantationn= 5 biological replicates.mQuantification of the proportion of the donor-derived cell in BM. **P= 0.0055,n= 4 biological replicates.nExpression ofNlrc3,Runx1,Il1b, and Notch-related genes in WT,Nlrc3−/−whole FL at E14.5 by qPCR. ns = 0.8168, *P= 0.0137, 0.0205, 0.0107, **P= 0.0078, 0.0039, 0.0063, ****P< 0.0001. Error bars, mean ± s.d., the exactp-values mentioned above are listed from left to right by using two-tailed, unpaired Student’st-test in (d,f,g,j,k,m,n). Illustrations created with BioRender.com. Source data are provided as a Source Data file. Reporting summary Further information on research design is available in the Nature Portfolio Reporting Summary linked to this article.